Dissipative binding of atoms by non-conservative forces The formation of molecules and supramolecular structures results from bonding by conservative forces acting among electrons and nuclei and giving rise to equilibrium configurations defined by minima of the interaction potential. Here we show that bonding can also occur by the non-conservative forces responsible for interaction-induced coherent population trapping. The bound state arises in a dissipative process and manifests itself as a stationary state at a preordained interatomic distance. Remarkably, such a dissipative bonding is present even when the interactions among the atoms are purely repulsive. The dissipative bound states can be created and studied spectroscopically in present-day experiments with ultracold atoms or molecules and can potentially serve for cooling strongly interacting quantum gases. In most experiments investigating coherent quantum dynamics, dissipation is an undesirable process. However, there have been several recent theoretical proposals for turning controlled dissipation into a useful resource, for example, for the realization of interesting many-body quantum states [1] , [2] , [3] , [4] . The main idea is to engineer the interaction with the environment such that the combination of coherent and dissipative dynamics drives the system in question to a stationary state identical to the quantum state of interest. The feasibility of such a reservoir engineering has already been demonstrated experimentally [5] . In our work, we employ a similar idea to show that a bond between two interacting atoms (or molecules) can be induced by dissipation, thereby extending the notion of a bonding mechanism from purely conservative to dissipative forces. The bond manifests itself as a stationary state of the scattering dynamics that confines the atoms at a fixed distance. Owing to the unprecedented control available for ultracold atoms and molecules [6] , the characteristics of the resulting molecules such as bond lengths and spectroscopic properties are highly tunable and can be observed in current experiments. As a specific physical implementation, we first consider two interacting atoms whose motion is restricted to one-spatial dimension (1D), see Fig. 1a . For ultracold atoms and molecules, such a constraint can be enforced by appropriate trapping potentials [6] . We assume the internal level structure of the atoms as shown in Fig. 1b : each has one internal state |1› exhibiting a distance-dependent interaction shift, and two other non-interacting states |2› and |3›, with |2› undergoing spontaneous decay into states |1› and |3›. This particular level structure is quite common in ultracold atoms and molecules, see the Methods section for two different possible realizations based on Rydberg-dressed atoms [7] , [8] , [9] or laser-cooled molecules [10] , [11] , [12] . Although our approach is general, we focus on dipole–dipole interactions, as this brings in additional tunability due to the anisotropy of the interaction potential [13] . We generalize our results to higher spatial dimensions and many-particle systems, and discuss the prospects of using dissipative bonding as a cooling mechanism for strongly interacting quantum gases. 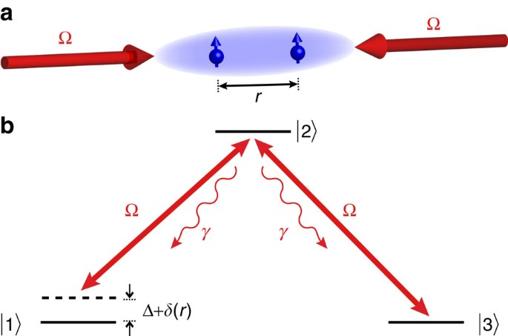Figure 1: Setup of the system. (a) Strong confinement by external fields restricts the atoms’ motion to one spatial dimension parallel to the two counter-propagating laser beams represented by the driving fields with Rabi frequencies Ω; (b) internal level structure of the atoms. Two internal statesandare coupled to a metastable statespontaneously decaying with a rateγ. The laser field coupling the statesandis detuned from the resonance by Δ; stateis subject to a dipolar interaction shiftδ(r), which depends on the interparticle distancer; statesandare non-interacting. Figure 1: Setup of the system. ( a ) Strong confinement by external fields restricts the atoms’ motion to one spatial dimension parallel to the two counter-propagating laser beams represented by the driving fields with Rabi frequencies Ω; ( b ) internal level structure of the atoms. Two internal states and are coupled to a metastable state spontaneously decaying with a rate γ . The laser field coupling the states and is detuned from the resonance by Δ; state is subject to a dipolar interaction shift δ ( r ), which depends on the interparticle distance r ; states and are non-interacting. Full size image Interaction-induced coherent population trapping The process behind the formation of the bond is coherent population trapping (CPT) [14] , [15] . In our setup, we include two counter-propagating laser beams; the one is resonant with the transition between states |2› and |3›, and another is detuned by Δ from the resonance between |1› and |3›; for simplicity we set the Rabi frequencies of both fields to Ω. CPT entails a dark state, that is, a stationary state that cannot absorb photons. For a system of two atoms subject to the electromagnetic field treated as a reservoir [16] , the dynamics is obtained from the quantum master equation, whose stationary solution is given by the condition d ρ /d t =0. Here H is the Hamiltonian describing the two atoms and their interaction with the laser fields, ρ is the density operator describing the two atoms, and γ n and c n are the rates and corresponding jump operators associated with spontaneous decay, see the Methods section for details. From the master equation (1), one can extract an effective non-Hermitian Hamiltonian, H eff = H − iV d , containing a dissipative potential, The zero-energy eigenstate of H eff corresponds to the dark state if its dissipation vanishes, that is, . In the non-interacting but resonant case, δ ( r )≡Δ=0, the dark state for each atom is given by . Taking the coupling to translation via the Doppler effect into account retains this dark state and gives rise to the well-known velocity-selective CPT [15] . In contrast, here we consider the regime where the kinetic energy is small compared with the dipolar interaction between the atoms, which in turn is small compared with both the laser driving and the decay, that is, . We note that although the conventional velocity-selective CPT scheme can preserve a dark state in presence of the dipole–dipole interactions between the ground and excited states [17] , our setup involves interactions only in state |1› and therefore does not entail a true dark state corresponding to zero dissipation. In the limit of infinite mass m , we find via perturbation theory, that the dissipation has a minimum when the atoms are separated by a distance r d where the dipolar interaction δ ( r ) destructively interferes with the detuning Δ the most, Here d is the dipole moment of state , ε 0 the vacuum permittivity, ħ Planck’s constant, and the numerical constants are and . The width of the Raman hole in the absorption profile, on the order of Ω 2 / γ , amounts to the distances where the dipolar interaction and the detuning approximately cancel each other. Although in conventional CPT schemes the photon-scattering rate depends quadratically on the detuning from the resonance, the dipolar interaction shift scales with distance as . This results in an anharmonic shape of the dissipative potential V d ( r ), and thereby in dependence of r d on the Rabi frequency Ω in equation (3). Even though there still is some residual dissipation for atoms confined to the vicinity of r d , the probability to find the atoms separated by r d is strongly enhanced. Such a confinement of the atoms amounts to the formation of a dissipative bond. Additional perturbations arising owing to a finite mass lead to a stationary state that exhibits a distribution of distances sharply centred around r d rather than a single-fixed distance. In the case of molecules bound by conservative forces, the strength of the bond is characterized by the binding energy—the amount of energy needed to be transfered to a molecule for dissociation. Similarly, the strength of the dissipative bond can be characterized by an imaginary binding energy, reflecting the amount of dissipation that is required to be added to the system in order to achieve dissociation. The imaginary binding energy is then defined as the difference between the decay rates at r =∞ and r = r d , and can be calculated in the regime Ω< γ as Numerical simulations of the dynamics We now turn to numerical simulations to confirm the existence of the dissipative bond. We solve the quantum master equation (1) using the wave-function Monte-Carlo method [18] , see the Methods section for details. During the time evolution the atomic positions are redistributed by the kinetic energy and photon recoil, and the atomic population is accumulated in the vicinity of r d on a fast timescale of a few tens of γ −1 . For an ensemble of atoms with randomly distributed initial conditions, we observe the appearance of a quasi-stationary distribution strongly peaked around r d , see Fig. 2 . For even longer times, the spatial distribution of the atoms appears to evolve towards a completely delocalized distribution of the laboratory-frame positions, r 1 and r 2 , compatible with a relative distance r d ≈500 nm. This constitutes evidence that in the long-time limit the state corresponding to the dissipative bond is a state with a relatively low entropy, which is confirmed by the semiclassical studies of the dynamics described below. Once the dissipative bond has been formed, it is possible to further reduce the probability of subsequent spontaneous decay events by decreasing the Rabi frequencies Ω. This leads to an effective decay rate γ eff = γp 2 , with p 2 the total probability of any of the atoms being in state |2›. For experimentally realistic parameters, see the Methods section for details, we find p 2 ≈0.01, implying the lifetime of the dissipative bond to be longer than the timescale of the formation of the bond. Furthermore, we find that the reduction of the Rabi frequencies does not lead to a significant increase of the spread about r d , and that lifetimes of the bound state exceeding can be achieved. 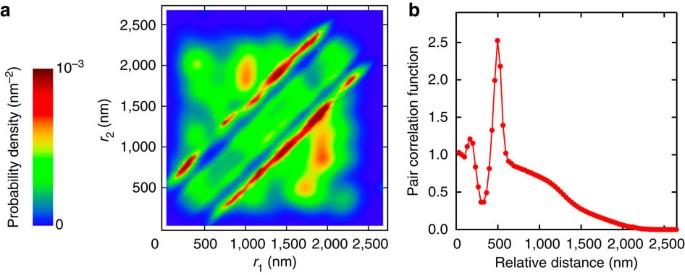Figure 2: Formation of the dissipatively bound states. (a) The probability density distribution shows that the absolute coordinates of the two particles,r1,r2, are delocalized; (b) the pair-correlation function exhibits a sharp peak aroundrd=500 nm. Parameters correspond to a pair of Rydberg-dressed caesium atoms (see the Methods section for details). Figure 2: Formation of the dissipatively bound states. ( a ) The probability density distribution shows that the absolute coordinates of the two particles, r 1 , r 2 , are delocalized; ( b ) the pair-correlation function exhibits a sharp peak around r d =500 nm. Parameters correspond to a pair of Rydberg-dressed caesium atoms (see the Methods section for details). Full size image The above results can be generalized to higher spatial dimensions, thereby allowing to study the motion of the bound atoms. This merely requires the inclusion of additional counter-propagating laser beams as used in conventional laser cooling setups [19] . For a two-dimensional (2D) configuration, we consider the case when the quantization axis defined by the electric dipole moment is perpendicular to the plane of the motion, that is, when the dipolar interaction is always repulsive. Then, the dissipative bond restricts the relative radial motion to a ring where the atoms are separated by r d . The effective Hamiltonian H eff for the remaining angular motion is then described by a 2D rigid rotor, , with J z the projection of the angular momentum on the quantization axis. The rotational constant can be widely tuned by changing r d ; for typical experimental realizations, we find that values of B ~100–1,000 Hz are realistic, that is, by far exceeding the effective decay rate γ eff . The rotational spectrum of the bound atoms can be then probed with standard techniques of molecular spectroscopy. In three-spatial dimensions (3D), the constrained relative motion of the two atoms is even richer due to the anisotropy of the dipolar interaction. The dynamics is confined to a surface defined by with θ the angle between the collinear dipoles and the interatomic radius-vector. Due to the rotational symmetry about the quantization axis, the projection of the angular momentum, J z , is conserved, allowing to reduce the problem to an effective one-dimensional problem. The effective potential corresponds to an azimuthally symmetric double well centred at θ =π/2, resulting in an almost equidistant spectrum consisting of tunnelling doublets, Fig. 3a , similar to those encountered in microwave spectra of ammonia [20] or molecules in strong laser fields [21] . 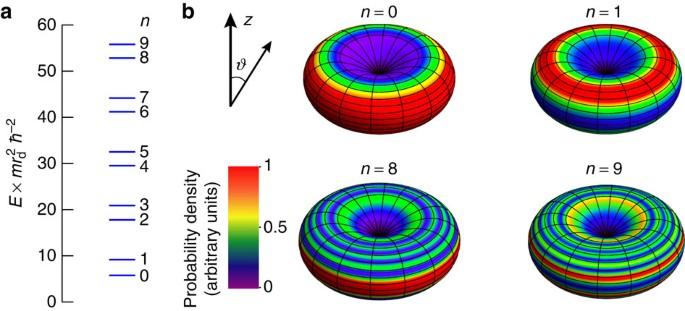Figure 3: Three-dimensional eigenstates. (a) The Lowest energy levels featuring tunnelling doublets due to the azimuthal symmetry of the interaction potential; (b) probability density distributions. The angleθgives the orientation of the collinear dipoles with respect to the vector connecting them. The quantum numberngives the number of nodes of the probability density distribution (purple colour) depending on the angleθ. The results shown correspond toJz=0. Figure 3b features the probability density distributions on the three-dimensional surface. Although the results shown in Fig. 3 correspond to J z =0, energy spectra and wavefunctions for other values of J z exhibit similar features. Figure 3: Three-dimensional eigenstates. ( a ) The Lowest energy levels featuring tunnelling doublets due to the azimuthal symmetry of the interaction potential; ( b ) probability density distributions. The angle θ gives the orientation of the collinear dipoles with respect to the vector connecting them. The quantum number n gives the number of nodes of the probability density distribution (purple colour) depending on the angle θ . The results shown correspond to J z =0. Full size image Experimental observation of the resulting bound states can be performed by making use of the techniques well-established in the area of ultracold quantum gases. In particular, a suitable setting would be a many-body system, in which the atoms are essentially uncorrelated at the beginning, with an average interatomic distance much larger than r d , so that many-body effects could be neglected. Then, the existence of the bound state will appear as a sharp peak in the pair-correlation function, see Fig. 2b , which is readily accessible through Bragg scattering [22] or noise correlation spectroscopy [23] , [24] . To analyse the behaviour in a many-body setting in more detail, we employ a semiclassical model of the dynamics, see the Methods section for the details. To compare this semiclassical approach with the quantum mechanical model, we calculated the pair-correlation function for the case of two particles in a one-dimensional trap, see Fig. 4a . Despite being obtained in different temperature regimes, there is a good agreement with the quantum mechanical treatment of Fig. 2b . The observed decrease in entropy towards a stationary value, shown in the inset of Fig. 4b , is a sign of a substantial cooling of the relative motion in the system. As shown in Fig. 4b,c , the appearance of a sharp peak around r d corresponding to the formation of dissipative bonds is independent of the number of particles and the dimensionality of the system. Note that in all the cases described above the density is low enough to neglect any effects beyond two-body interactions. 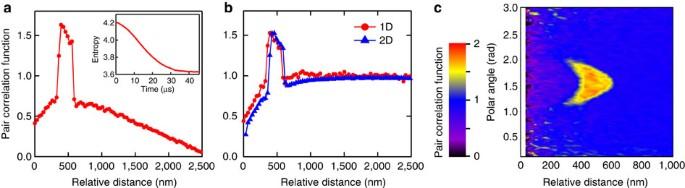Figure 4: Semiclassical simulations of the dynamics. (a) Pair correlation of two particles in 1D, using the same parameters as inFig. 2. The inset shows the time evolution of the relative distance entropy. (b) Many-body systems containing 102particles in 1D (red circles) and 104particles in 2D (blue triangles). (c) 104particles in 3D, with the polar angleθas shown inFig. 3b. Figure 4: Semiclassical simulations of the dynamics. ( a ) Pair correlation of two particles in 1D, using the same parameters as in Fig. 2 . The inset shows the time evolution of the relative distance entropy. ( b ) Many-body systems containing 10 2 particles in 1D (red circles) and 10 4 particles in 2D (blue triangles). ( c ) 10 4 particles in 3D, with the polar angle θ as shown in Fig. 3b . Full size image We have established the existence of a dissipative-binding mechanism triggered by non-conservative forces found in interaction-induced coherent-population trapping. Our results are applicable to a large class of atomic and molecular systems, while the properties of the bound states are highly tunable. Finally, we note that the mechanism underlying the formation of the dissipative bond can potentially be used for cooling of strongly interacting many-body systems. Clearly, the appearance of a low-entropy stationary state independent of the initial conditions already amounts to a demonstration of a cooling of the relative motion. In the high-density regime, the correlation length r d will be modified by an effective coordination number, embodying the interactions of an individual atom with its surroundings in the stationary state. Despite this renormalization, the formation of dissipatively bound complexes [25] in free space or even the realization of dipolar crystals [26] , [27] appear possible. Quantum dynamics The coherent part of the dynamics according to the quantum master equation (1), is given by the two-atom Hamiltonian, Here i =1,2 and k label the atoms and their corresponding momentum states, and is the Fourier transform of the dipole–dipole interaction potential. The dissipative part of equation (1) contains the rates γ n = γ and jump operators in the Lindblad form, responsible for the decay of each atom from state |2›. The index i n =1,2 runs over the two atoms, while j n =1,3 accounts for the two final states, and Δ k n contains all possible values of the emitted photon’s wave vector [18] . The results presented in Fig. 2 correspond to a state after the evolution time of 4.6 μs, averaged over 250 realizations with random initial conditions. In each realization, two atoms are confined in a one-dimensional box , which corresponds to the three-dimensional particle density of 3 × 10 11 cm −3 . The initial state was chosen as a quasi-thermal distribution of Gaussian wavepackets having an initial momentum of 4 ħk r , where k r is the recoil momentum. Semiclassical dynamics For the semiclassical analysis, we use Langevin equations for the motion of the particles. In analogy to the semiclassical description of laser cooling [28] , we introduce a velocity-dependent friction force and a stochastic heating force, which are derived within perturbation theory. In addition, our model includes a transition rate to a bound channel, , in which two bound particles move with the same velocity. This binding term is only active for particles separated by | r − r d |< w d , where w d is corresponds to the half-width at half-maximum of the absorption profile. The reverse process, responsible for breaking of the dissipative bond, is governed by the stochastic heating force mentioned above. All results shown in Fig. 4 were obtained using the same atomic parameters and density as in the quantum treatment, with the pair correlations computed at a time of 4.6 μs. As the semiclassical approach is only valid for momenta much larger than ħk r [28] , the initial momentum distribution was chosen from a Boltzmann distribution with . The relative distance entropy was calculated as the Shannon entropy , where p ( r i ) gives a probability to find atoms separated by distance r i in the box. Experimental implementation We consider two different realizations of our setup depicted in Fig. 1 , based on driven-dissipative Rydberg atoms [29] , [30] , [31] and laser-cooled molecules. In the case of Rydberg-dressed caesium atoms, the states |1› and |3› are chosen as different hyperfine components of the electronic ground state, 6 2 S 1/2 , of caesium. The state |1› is provided with a dipole moment of d =15 D perpendicular to the 1D trap due to Rydberg dressing in an external electric field [7] , [8] , [9] ; laser fields Ω= γ /4 drive the 6 2 S 1/2 → 6 2 P 3/2 transition having a linewidth of γ =2 π × 5.2 MHz. These parameters correspond to an imaginary binding energy of E b = i 2π ħ × 31 kHz. We would like to stress that in contrast to the previous Rydberg dressing proposals for the observation of interactions in a Bose–Einstein condensate, the requirements on coherence times for the observation of the dissipative bond are much less stringent; preserving coherence on the timescale of the rotational constant B ~100 Hz can be achieved in present-day experiments [32] , [33] , [34] , [35] , [36] , [37] , see Löw et al. [38] for a recent review. Although we exemplified our scheme by the case of bonding between a pair of atoms, it is equally applicable to bonding between a pair of molecules, such as strontium monofluoride (SrF) that is being laser-cooled [11] . For SrF, different hyperfine components, F =0, 1, of the X 2 Σ + ( v =0; N =1, J =1/2) state are chosen as |1› and |3›. Here a dipole moment of 3.5 D in the rotating frame is imprinted on via microwave dressing [39] , while the fields Ω= γ /4 drive transitions to the electronically excited A 2 Π 1/2 ( v ′=0; N =0, J ′=1/2) whose natural linewidth is γ =2 π × 7 MHz. How to cite this article: Lemeshko, M. & Weimer, H. Dissipative binding of atoms by non-conservative forces. Nat. Commun. 4:2230 doi: 10.1038/ncomms3230 (2013).